Sensitivity control through attenuation of signal transfer efficiency by negative regulation of cellular signalling Sensitivity is one of the hallmarks of biological and pharmacological responses. However, the principle of controlling sensitivity remains unclear. Here we theoretically analyse a simple biochemical reaction and find that the signal transfer efficiency of the transient peak amplitude attenuates depending on the strength of negative regulation. We experimentally find that many signalling pathways in various cell lines, including the Akt and ERK pathways, can be approximated by simple biochemical reactions and that the same property of the attenuation of signal transfer efficiency was observed for such pathways. Because of this property, a downstream molecule should show higher sensitivity to an activator and lower sensitivity to an inhibitor than an upstream molecule. Indeed, we experimentally verify that S6, which lies downstream of Akt, shows lower sensitivity to an epidermal growth factor receptor inhibitor than Akt. Thus, cells can control downstream sensitivity through the attenuation of signal transfer efficiency by changing the expression level of negative regulators. The sensitivities of upstream and downstream molecules to an activator or inhibitor can differ, and variations in sensitivity among cell lines are also observed. Such sensitivity is often measured using the peak amplitude [1] , [2] , [3] , [4] , [5] , equilibrium amplitude [6] , [7] , [8] , [9] , duration [10] , [11] , [12] and integration (the area under a curve) [13] , [14] , [15] of the activity of a signalling molecule. Sustained amplitude at equilibrium has been well characterized and studied, and several possible mechanisms for controlling the sensitivity of the equilibrium amplitude have been proposed, such as substrate depletion in a biochemical reaction [16] , [17] , [18] and the characteristics of network motifs [6] , [10] , [19] , [20] . However, the peak amplitude of transient response has not been well characterized. Importantly, under physiological conditions, transient response is one of the characteristics of dynamic cellular behaviour. For example, when the peak amplitude of an input to a bistable system exceeds a threshold value, cellular response is turned on [21] , [22] . In addition, the peak amplitudes of transient response are very important because they are often used as an index of signalling activity in experiments that include western blotting. However, the mechanism responsible for controlling the sensitivity of the peak amplitude remains to be elucidated. We previously found that weak, sustained epidermal growth factor receptor (EGFR) phosphorylation, rather than strong, transient phosphorylation, strongly induced the phosphorylation of S6, a downstream molecule in the Akt pathway. This result indicates that the peak amplitudes of transient and sustained time courses between upstream and downstream molecules can be decoupled in PC12 cells in response to EGF stimulation ( Fig. 1a ) [23] . Interestingly, a consecutive first-order reaction (also known as a leaky integrator [22] or a low-pass filter [23] ), which represents a simple signalling pathway, can reproduce this decoupling effect [23] . Even in the same pathway, the upstream and downstream signals couple or do not couple, depending on the temporal pattern of the upstream signals ( Fig. 1a ). This dependence suggests that the attenuation of the signal transfer efficiency of the peak amplitudes depends on the temporal pattern of upstream signals, and that the attenuation is responsible for the decoupling effect. Thus, the mechanism leading to the attenuation of the signal transfer efficiency remains to be elucidated. 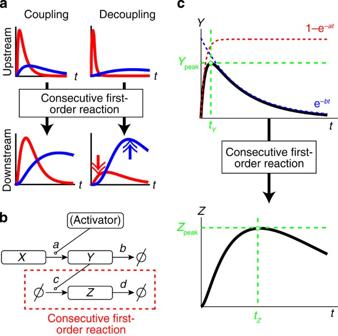Figure 1: Activator model. (a) Time courses of the activities of the upstream and downstream molecules under either coupling or decoupling conditions. (b) The boxes and arrows represent the molecules and their chemical reactions, respectively. A circle with a line through it represents a pool of substrates or degradation products. A circle connected to an arrow represents a catalytic contribution to the reaction. The constantsa,b,canddindicate the rate constants of the respective reactions. (c) Representative time courses ofYandZ(black lines).YpeakandZpeakare the peak amplitudes of the time courses ofYandZ, respectively.tYandtZare the peak times of the time courses ofYandZ, respectively. The coloured dashed lines in the upper panel are the asymptotic lines of the time course ofY. The rate constantsaandbalso represent the synthesis and decay rates of the time course ofYwhenais larger thanb. Figure 1: Activator model. ( a ) Time courses of the activities of the upstream and downstream molecules under either coupling or decoupling conditions. ( b ) The boxes and arrows represent the molecules and their chemical reactions, respectively. A circle with a line through it represents a pool of substrates or degradation products. A circle connected to an arrow represents a catalytic contribution to the reaction. The constants a , b , c and d indicate the rate constants of the respective reactions. ( c ) Representative time courses of Y and Z (black lines). Y peak and Z peak are the peak amplitudes of the time courses of Y and Z , respectively. t Y and t Z are the peak times of the time courses of Y and Z , respectively. The coloured dashed lines in the upper panel are the asymptotic lines of the time course of Y . The rate constants a and b also represent the synthesis and decay rates of the time course of Y when a is larger than b . Full size image In this study, we first examined the conditions for the attenuation of signal transfer efficiency in a consecutive first-order reaction and found that it depended on the relationship between the duration of upstream signal and the time constant of negative regulation. We experimentally found that considerable numbers of signalling pathways in various cell lines, including the Akt and ERK pathways, can be reasonably approximated by a consecutive first-order reaction, although actual molecular networks should consist of multiple complex biochemical reactions, and that the property of attenuation of signal transfer efficiency is conserved among such pathways. These findings led us to observe that the attenuation of signal transfer efficiency controls the sensitivities to an activator or an inhibitor, and that the alteration of sensitivity can be controlled through negative regulation. We experimentally verified the control of sensitivity to an inhibitor in the Akt pathway. Our study demonstrates that the attenuation of signal transfer efficiency through negative regulation is a conserved property of the signalling pathway, and is one of the core mechanisms of controlling the sensitivity to an activator and an inhibitor. This result indicates that cells can control sensitivity to an activator or an inhibitor by changing the expression level of negative regulators. Attenuation of the signal transfer efficiency We constructed a simple model using a consecutive first-order reaction ( Fig. 1b ; see Supplementary Note 1 ) and numerically analysed the conditions for the attenuation of signal transfer efficiency. The model can be described using the following ordinary differential equations: The initial conditions were given as follows: and the analytical solution of the equations is where ( a ≠ b ≠ d ). Y and Z were regarded as the amounts of activated upstream and downstream molecules of a signalling pathway, respectively. In this study, we focused on the relationships between Y and Z ; therefore, the biological counterpart of X was not specified. The model had four rate constants: a , b , c and d . The constant a is the synthesis rate constant of Y , and the value of a simultaneously means the concentration of the activator. The constant b is the degradation rate constant of Y . The constant c is the synthesis rate constant of Z . The constant d is the degradation rate constant of Z . The degradation of Z can be regarded as a negative regulation of the pathway from Y to Z ; therefore, the value of d corresponds to the strength of negative regulation. Hereafter, this model is referred to as the activator model. The time course of Y exhibited a single peak and was expressed as the sum of two exponential functions ( Fig. 1c ). The rate constants a and b represented the synthesis and decay rates of the time course of Y . The time course of Z also exhibited a single peak. Hereafter, the peak amplitudes of Y and Z are referred to as Y peak and Z peak , respectively, and the peak times of Y and Z are referred to as t Y and t Z , respectively. We altered the time course of Y by changing a and b , and examined the response of Z peak . Note that the amplitude of Z was uniformly scaled by k (= c / d , see Supplementary Note 1 ); therefore, the ratio of Z peak to Y peak was also scaled by k . To remove the effect of k , the signal transfer efficiency E was defined by the following normalized form: Note that as d increases , Z peak decreases, and the ratio of Z peak to Y peak also decreases. However, E increases because 1/ k (= d / c ) increases along with the increase of d and because the increase of 1/ k overcomes the decrease of Z peak. We examined how the signal transfer efficiency E is determined using numerical simulation ( Fig. 2 ). The Z peak indicated in red became lower than that indicated in blue, despite exhibiting the same Y peak ( Fig. 2a ), indicating that the Y signal (shown in red) was not transferred efficiently to Z compared with the signal indicated in blue. We next examined the effects of parameters a and b on Y peak and Z peak ( Fig. 2b,c ). Y peak was determined by the ratio of a to b ( a / b ) and increased as a function of a / b ( Supplementary Fig. S1 ). Similarly, Z peak seemed to be determined by a / b when both a and b were smaller than d ( Fig. 2c ). However, Z peak seemed to become independent of a / b and instead was determined by b when a was larger than d . We confirmed that similar results were obtained for a wide range of d values ( Supplementary Fig. S1 ). We then obtained the signal transfer efficiency E from Z peak and Y peak ( Fig. 2d ). E reached a maximum value of ∼ 1 when a or b was smaller than d , and decreased to values <1 when either a or b was larger than d . This finding indicates that the signal transfer efficiency E was higher when either the synthesis or the degradation rate constant of the upstream signal was smaller than the rate constant of negative regulation, whereas E was attenuated when both the synthesis and degradation rate constants of the upstream signal became larger than the rate constant of negative regulation. 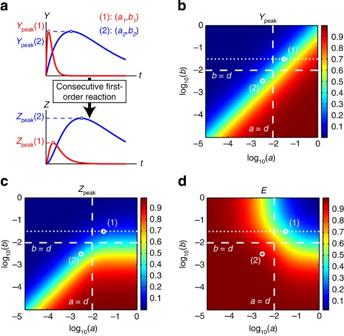Figure 2: Attenuation of signal transfer efficiency. (a) The degree of attenuation depends on the upstream time course. The time courses ofY, indicated in red and blue, have different parameters. (b) Dependence ofYpeakonaandb. The colour scale indicatesYpeak. The values ofcanddwere set at 0.01. The white circles correspond to the time courses shown in panela. The white dashed lines indicate whenaorbequalsd. The white dotted line corresponds to the red line inFig. 3a. (c) Dependence ofZpeakonaandb. (d) Dependence ofEonaandb. Figure 2: Attenuation of signal transfer efficiency. ( a ) The degree of attenuation depends on the upstream time course. The time courses of Y , indicated in red and blue, have different parameters. ( b ) Dependence of Y peak on a and b . The colour scale indicates Y peak . The values of c and d were set at 0.01. The white circles correspond to the time courses shown in panel a . The white dashed lines indicate when a or b equals d . The white dotted line corresponds to the red line in Fig. 3a . ( c ) Dependence of Z peak on a and b . ( d ) Dependence of E on a and b . Full size image We also obtained analytical solutions for Y peak and Z peak (see Supplementary Note 1 ). An analytical solution for Y peak (and also for t Y ) can be easily obtained, but it is not easy to obtain an analytical solution for Z peak . We divided the parameter space into three areas (areas I–III, Supplementary Fig. S2 ) and approximated the analytical solution of Z to obtain the approximate analytical solution of Z peak and t Z . Z peak in the approximate analytical solution ( Supplementary Fig. S2 ) was very similar to Z peak in the numerical solution ( Fig. 2c ), except for some inaccurate approximations in a few areas ( Supplementary Fig. S2 ). On the basis of the approximate analytical solutions, we obtained the conditions under which decoupling occurs using simple expressions (see Supplementary Table S1 ). This result indicates that the decoupling effect was caused by the strong attenuation in the signal transfer efficiency, E . Attenuation of the efficiency is a conserved property We attempted to validate the signal transfer efficiency experimentally. For this purpose, we determined how to estimate E experimentally ( Fig. 3 ; Supplementary Fig. S3 ). We found that E can be estimated by the duration ( t 1/2 ) of the upstream signal and the time constant τ ( τ =1/ d ) of negative regulation of a signalling pathway, both of which can be experimentally measured ( Fig. 3a ; Supplementary Fig. S3 ). E was attenuated when t 1/2 became shorter, and E was approximately equal to 0.5 when t 1/2 was equal to τ ( Supplementary Fig. S3 ), indicating that the attenuation of E depends on the ratio of t 1/2 to τ . Therefore, E can be controlled by negative regulation. The theoretical estimate of E against t 1/2 normalized by τ in the model ( Fig. 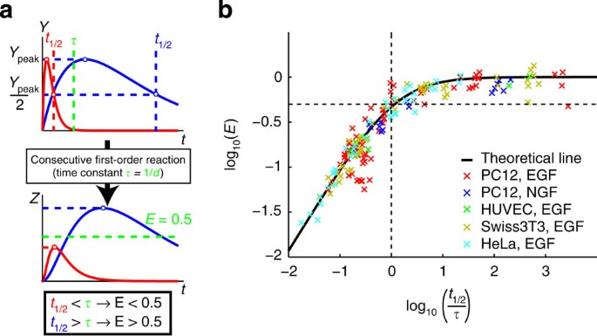Figure 3: Attenuation of the signal transfer efficiency is a conserved property. (a) The duration of upstream signal,t1/2, is the time at which the value ofYhas decreased to half of the value ofYpeak. The time constantτis the inverse of the rate constant,d, of the negative regulation of the consecutive first-order reaction. Ift1/2is shorter thanτ, thenEbecomes <0.5, whereas ift1/2is longer thanτ, thenEbecomes >0.5. (b) A plot ofEagainstt1/2, normalized byτ. The solid line indicates the theoretical line of the model, which is given by(seeSupplementary Fig. S3). The crosses indicate experimental values ofE. The horizontal and vertical dashed lines indicate whereE=0.5 andt1/2=τ, respectively. 3b , solid line) was calculated using Figure 3: Attenuation of the signal transfer efficiency is a conserved property. ( a ) The duration of upstream signal, t 1/2 , is the time at which the value of Y has decreased to half of the value of Y peak . The time constant τ is the inverse of the rate constant, d , of the negative regulation of the consecutive first-order reaction. If t 1/2 is shorter than τ , then E becomes <0.5, whereas if t 1/2 is longer than τ , then E becomes >0.5. ( b ) A plot of E against t 1/2 , normalized by τ . The solid line indicates the theoretical line of the model, which is given by (see Supplementary Fig. S3 ). The crosses indicate experimental values of E . The horizontal and vertical dashed lines indicate where E =0.5 and t 1/2 = τ , respectively. Full size image E is approximately half of its maximal value when t 1/2 is equal to τ . If t 1/2 is shorter than τ , then E is <0.5 whereas if t 1/2 is longer than τ , then E is >0.5 ( Fig. 3a ). For example, consider a pathway where τ is 30 min. If t 1/2 is 10 min (shorter than τ ), then E is smaller (0.23). Conversely, if t 1/2 is 60 min (longer than τ ), then E is larger (0.62). This result indicates that the signal transfer efficiency E attenuates when t 1/2 is shorter than τ . To examine whether the attenuation of the signal transfer efficiency is a general property of a signalling pathway, we measured the time courses of various signalling pathways by changing the doses of different ligands in various cell lines. Experimentally, E can be obtained under conditions where the time course of upstream molecules can be approximated by the sum of two exponential curves, and the pathway can be approximated by a consecutive first-order reaction ( Fig. 1c ). Among 568 sets of upstream and downstream time courses of signalling pathways ( Supplementary Data 1 ), 169 sets satisfied the conditions (see Supplementary Data 2 ; see also Methods and Supplementary Note 1 ), including the pAkt to pS6 pathway [23] . It is quite surprising that, although actual molecular networks should consist of multiple complex biochemical reactions, a considerable number of sets of time courses between upstream and downstream molecules (169 of 568 sets) can be reasonably approximated by simple linear reactions. This result suggests that, at a time resolution of minutes, the selected signalling pathways apparently behave as a simple linear input–output relationship, despite the reactions being more complex and nonlinear in reality. This result also suggests that, even if detailed information about reaction steps or schemes is unknown for a particular signalling pathway, a consecutive first-order reaction can potentially approximate the behaviours of considerable numbers of signalling pathways. Among the 169 sets studied, we first examined whether any attenuation of signal transfer efficiency was observed in PC12 cells for EGF-dependent pathways involving EGFR, Akt, ERK1, ERK2, S6 kinase, S6, eIF4B, RSK and c-Fos (70 sets of time courses in 16 pathways; see Supplementary Data 2 ). For such pathways, the experimental values of E lay along the theoretical line in the model ( Fig. 3b , red points). Therefore, E does indeed depend on the ratio of t 1/2 to τ, regardless of the pathway, and the attenuation property was conserved among these signalling pathways. We also asked whether this property is specific to EGF or whether it can be seen in other ligands, such as nerve growth factor (NGF). The values of E for the NGF-dependent signalling pathways in PC12 cells (six sets of time courses in two pathways) similarly lay along the theoretical line ( Fig. 3b , blue points; Supplementary Data 2 ). Thus, the attenuation property was conserved among the ligands. We also asked whether this property is specific to PC12 cells or whether it can be seen in other cell lines, such as human umbilical vein endothelial cells (HUVECs), Swiss 3T3 and HeLa cells. The values of E for the EGF-dependent signalling pathways in HUVECs (15 sets of time courses in 4 pathways; Fig. 3b , green points; Supplementary Data 2 ), Swiss 3T3 (39 sets of time courses in 12 pathways; Fig. 3b , yellow points; Supplementary Data 2 ) and HeLa (34 sets of time courses in 14 pathways; Fig. 3b , cyan points; Supplementary Data 2 ) similarly lay along the theoretical line. This result indicates that the attenuation property was conserved among the cell lines. In short, the attenuation of signal transfer efficiency seems to be a general property of all signalling pathways that can be approximated by a consecutive first-order reaction and is not specific to particular signalling pathways, ligands or cell lines. Control of sensitivity to an activator We found that the attenuation of the signal transfer efficiency depends on the temporal pattern of Y in a manner that further depends on the concentration of the activator (the concentration is represented by the rate constant a ). This result suggests that the attenuation of the signal transfer efficiency may cause a difference in the sensitivities of the upstream and downstream molecules to the activator. Therefore, we examined the effective dose of the activator for Y peak and Z peak ( Fig. 4 ). Note that a can be regarded as the concentration of the activator ( Fig. 4a,b ). Y peak increased as a became larger ( Fig. 4c , upper panel). For example, Y peak was 0.5 at a =0.0577, which is the half-maximal effective concentration of the activator (EC 50 ) for Y peak , and Y peak was 1 at a =100 (when d was 0.01). On the contrary, t 1/2 became smaller when a became larger. As we had already found that the signal transfer efficiency is attenuated as t 1/2 became smaller ( Fig. 3b ), the signal transfer efficiency was also attenuated as a became larger. Therefore, the value of E at a =0.0577 should be larger than that at a =100 ( Fig. 4c , middle panel). Because Z peak was relative to the product of Y peak and E , the value of Z peak at a =0.0577 should be larger than half of the value of Z peak at a =100. Thus, the EC 50 for Z peak became smaller than that of Y peak ( Fig. 4c , lower panel). This relationship indicates a leftwards shift of the dose–response curve of Z peak compared with that of Y peak against a ( Fig. 4d ), which indicates that Z peak is more sensitive to an activator than Y peak . Thus, the attenuation of the signal transfer efficiency increased downstream sensitivity to an activator under the experimental conditions. Because the attenuation of the signal transfer efficiency is controlled by negative regulation, we examined the effect of negative regulation on the increase in downstream sensitivity. We defined an index of increase in downstream sensitivity, S i , as the ratio of the EC 50 for Y peak to the EC 50 for Z peak ( Fig. 4e ; Supplementary Fig. S4 ). A larger value of S i represents an increase in the sensitivity of Z peak compared with that of Y peak . S i decreased and became close to 1 when d became larger but never became <1, indicating that the EC 50 values for the upstream and downstream molecules became the same and that the upstream molecule never became more sensitive to the activator than the downstream molecule in the consecutive first-order reaction. S i became larger when d became smaller, indicating that the increase in the downstream sensitivity became larger as the rate constant of the negative regulation of the consecutive first-order reaction, d , became smaller. This result indicates that the downstream molecule is generally more sensitive to an activator than the upstream molecule under these conditions, and that the increase in the downstream sensitivity depends on the negative regulation. We confirmed these results using mathematical analysis ( Supplementary Fig. S4 and Supplementary Note 1 ). 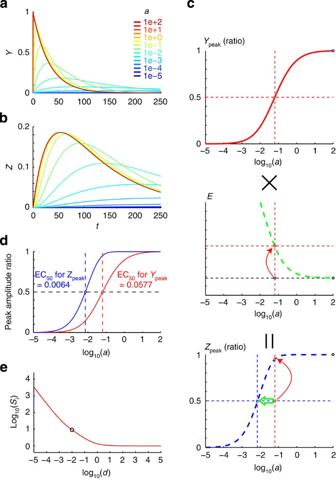Figure 4: The downstream molecule is more sensitive to an activator than the upstream molecule. (a,b) Time courses ofY(a)andZ(b)in response to the indicated values ofa(see inset). Note thatacan be regarded as the concentration of the activator. The values ofb,canddwere 0.03, 0.01 and 0.01, respectively. (c) Plots ofYpeak,EandZpeakagainsta. The attenuation ofEwas derived from panelaandFig. 3b,and it results in the decrease of EC50forZpeak. The maximal values ofYpeakandZpeakwere normalized to 1. (d) Dose–response curves ofYpeak(red line) andZpeak(blue line) to the activator. The lines correspond to the white dotted line inFig. 2b,c, and the values ofb,canddwere the same as those in panela. The coloured dashed lines indicate the EC50values forYpeakandZpeak. (e)Si(=EC50forYpeak/EC50forZpeak) is shown for the indicated values ofd. The circle indicates the parameters fora–d. Figure 4: The downstream molecule is more sensitive to an activator than the upstream molecule. ( a , b ) Time courses of Y (a) and Z (b) in response to the indicated values of a (see inset). Note that a can be regarded as the concentration of the activator. The values of b , c and d were 0.03, 0.01 and 0.01, respectively. ( c ) Plots of Y peak , E and Z peak against a . The attenuation of E was derived from panel a and Fig. 3b, and it results in the decrease of EC 50 for Z peak . The maximal values of Y peak and Z peak were normalized to 1. ( d ) Dose–response curves of Y peak (red line) and Z peak (blue line) to the activator. The lines correspond to the white dotted line in Fig. 2b,c , and the values of b , c and d were the same as those in panel a . The coloured dashed lines indicate the EC 50 values for Y peak and Z peak . ( e ) S i (=EC 50 for Y peak /EC 50 for Z peak ) is shown for the indicated values of d . The circle indicates the parameters for a – d . Full size image Control of sensitivity to an inhibitor Next, we examined the sensitivity to an inhibitor. We created an inhibitor model by adding an inhibitor to the activator model while maintaining the same relationship between Y and Z ( Fig. 5a ; see Supplementary Note 1 ). 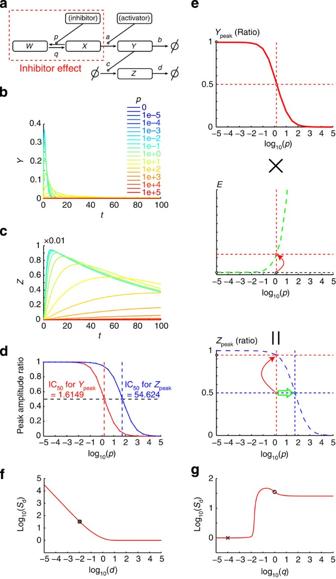Figure 5: The downstream molecule is less sensitive to an inhibitor than the upstream molecule. (a) Inhibitor model. The inhibitor acts onX, thereby inhibiting the activation ofY. The notations are the same as those used inFig. 1b. (b,c) Time courses ofY(b) andZ(c) in response to the indicated values ofp(see inset). Note thatpcan be regarded as the concentration of the inhibitor. The values fora,b,c, dandqwere set at 1, 1, 0.01, 0.01 and 1, respectively. The inhibitor was administered and reached equilibrium before stimulation. (d) Dose–response curves ofYpeak(red line) andZpeak(blue line) for the inhibitor. The dashed lines indicate the IC50values forYpeakandZpeak. The maximal values ofYpeakandZpeakwere normalized to 1. (e) Plots ofYpeak,EandZpeakagainstp. The attenuation ofEwas derived from panelbandFig. 3b, and results in the increase of IC50forZpeak. (f,g)Sd(=IC50forZpeak/IC50forYpeak) is shown for the indicated values ofdandq, respectively. The remaining parameters were the same as those used in panelsb–e. The black circle and the cross indicate the parameters used inFig. 5and inSupplementary Fig. S6, respectively. The model can be described using the following ordinary differential equations: Figure 5: The downstream molecule is less sensitive to an inhibitor than the upstream molecule. ( a ) Inhibitor model. The inhibitor acts on X , thereby inhibiting the activation of Y . The notations are the same as those used in Fig. 1b . ( b,c ) Time courses of Y ( b ) and Z ( c ) in response to the indicated values of p (see inset). Note that p can be regarded as the concentration of the inhibitor. The values for a , b , c, d and q were set at 1, 1, 0.01, 0.01 and 1, respectively. The inhibitor was administered and reached equilibrium before stimulation. ( d ) Dose–response curves of Y peak (red line) and Z peak (blue line) for the inhibitor. The dashed lines indicate the IC 50 values for Y peak and Z peak . The maximal values of Y peak and Z peak were normalized to 1. ( e ) Plots of Y peak , E and Z peak against p . The attenuation of E was derived from panel b and Fig. 3b , and results in the increase of IC 50 for Z peak . ( f,g ) S d (=IC 50 for Z peak /IC 50 for Y peak ) is shown for the indicated values of d and q , respectively. The remaining parameters were the same as those used in panels b – e . The black circle and the cross indicate the parameters used in Fig. 5 and in Supplementary Fig. S6 , respectively. Full size image We then examined the effect of the prior addition of the inhibitor on Y peak and Z peak in response to a fixed value of a (a fixed concentration of an activator; Fig. 5 ). The model has two new rate constants, p and q ; these constants are the binding and dissociation rate constants of the inhibitor with respect to X , respectively. The value of p simultaneously means the concentration of the inhibitor. We assumed that the inhibitor was administered and reached equilibrium before stimulation, and we set the initial conditions as follows: Hereafter, this model is referred to as the inhibitor model. Both Y peak and Z peak decreased as p increased ( Fig. 5b,c ). The half-maximal effective concentration of the inhibitor (IC 50 ) for Y peak was 1.61, and the value for Z peak was 54.6 ( Fig. 5d ). In other words, Z peak was less sensitive to the inhibitor compared with Y peak . Similar to EC 50 , t 1/2 became smaller when p became smaller. As previously found, the signal transfer efficiency attenuates as t 1/2 becomes smaller ( Fig. 3b ); therefore, E also is attenuated as p becomes smaller. Therefore, the value of E at p =1.61 should be larger than that at p =10 −5 ( Fig. 5e , middle panel). Because Z peak was relative to the product of Y peak and E , Z peak at p =1.61 should be larger than half the value of Z peak at p =10 −5 . Thus, the IC 50 for Z peak became larger than that of Y peak ( Fig. 5e , lower panel). This result indicates that the attenuation of the signal transfer efficiency decreased downstream sensitivity to an inhibitor. Thus, the attenuation of signal transfer efficiency is a core mechanism of the decrease in the downstream sensitivity to an inhibitor. We defined an index of decreasing sensitivity, S d , as the ratio of the IC 50 for Z peak to the IC 50 for Y peak ( Supplementary Fig. S5 ) and examined the effect of negative regulation on the decrease in downstream sensitivity to an inhibitor. A larger value of S d represents a larger decrease in the sensitivity of Z peak compared with that of Y peak . S d never became <1 within the indicated parameter space ( Supplementary Fig. S5 ), indicating that the downstream sensitivity to an inhibitor was always lower than the upstream sensitivity. S d became larger when d became smaller ( Fig. 5f ; Supplementary Fig. S5 ), indicating that the decrease in the downstream sensitivity is regulated by negative regulation and that the downstream molecule is generally less sensitive to an inhibitor than the upstream molecule under the given conditions. S d also became smaller when the dissociation rate constant of the inhibitor, q , became relatively small ( Fig. 5g ; Supplementary Fig. S5 ). Because an irreversible inhibitor can be regarded as a molecule with a very small dissociation rate constant, this finding suggests that the decrease in downstream sensitivity would be suppressed if an irreversible inhibitor were used. Indeed, the IC 50 for Z peak was the same as the IC 50 for Y peak when q was smaller than the value used in Fig. 5b,c ( Fig. 5g ; Supplementary Fig. S6 ). The decrease in the downstream sensitivity was suppressed when d was larger than q and when these parameters were relatively small ( Supplementary Fig. S5 ). These conditions for the suppression of a decrease in the downstream sensitivity were not affected by the other parameters, such as a and b , although S d did depend on these parameters ( Supplementary Fig. S5 ), indicating that the relationship between d and q is an essential and robust index for the suppression of a decrease in the downstream sensitivity. Thus, these results indicated that the downstream molecule was less sensitive to an inhibitor than the target molecule. Furthermore, we tried to verify experimentally that the downstream molecule was less sensitive to an inhibitor than the upstream molecule. We previously reported that the EGF-dependent Akt–S6 pathway can be approximately represented as a consecutive first-order reaction [23] . We used lapatinib, an EGFR inhibitor [9] , and measured the EGF-dependent phosphorylation of Akt and S6 in PC12 cells in the presence of the indicated concentrations of lapatinib ( Fig. 6a,b , respectively). Lapatinib inhibited the phosphorylation of both Akt and S6 in a dose-dependent manner. The IC 50 for the peak amplitude of the phosphorylation of Akt in response to lapatinib was ∼ 112 nM, and the value for S6 was ∼ 463 nM, which was ∼ 4.1 times higher than that of Akt ( Fig. 6c,d ). Thus, the downstream molecule did seem to be less sensitive to the inhibitor than the upstream molecule in the consecutive first-order reaction. We confirmed that these experimental data were reasonably reproduced by the inhibitor model ( Supplementary Fig. S7 ). 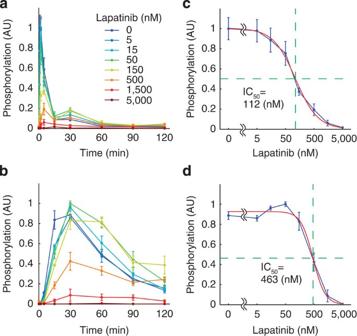Figure 6: Experimental validation of the decrease in the downstream sensitivity to an inhibitor. (a,b) After treatment with the indicated concentrations of lapatinib (an EGFR inhibitor) for 16 h, PC12 cells were stimulated with EGF (30 ng ml−1), and the phosphorylation levels of Akt and S6, respectively, were measured. The means and s.e.m. of three independent experiments are shown. (c,d) Dose–response curves of the peak amplitudes of phosphorylated Akt and S6, respectively. The experimental data (blue line) were fitted using a sigmoid curve (red line). The green dashed lines indicate the IC50values for the phosphorylated Akt and S6. Figure 6: Experimental validation of the decrease in the downstream sensitivity to an inhibitor. ( a,b ) After treatment with the indicated concentrations of lapatinib (an EGFR inhibitor) for 16 h, PC12 cells were stimulated with EGF (30 ng ml −1 ), and the phosphorylation levels of Akt and S6, respectively, were measured. The means and s.e.m. of three independent experiments are shown. ( c,d ) Dose–response curves of the peak amplitudes of phosphorylated Akt and S6, respectively. The experimental data (blue line) were fitted using a sigmoid curve (red line). The green dashed lines indicate the IC 50 values for the phosphorylated Akt and S6. Full size image The addition of an inhibitor before stimulation with an activator ( Figs 5 and 6 ) is the usual protocol for cell culture experiments in vitro ; however, the addition of an inhibitor after constitutive activation by an activator reflects more physiologically relevant in vivo situations, such as the administration of an anticancer drug to cancer cells expressing a constitutively active oncogene product. It is known that the mutation of an oncogene can result in the constitutive activation of a signalling pathway without a ligand, which leads to carcinogenesis. Therefore, we constructed an in vivo inhibitor model ( Supplementary Fig. S8 ) that mimics the effect of an inhibitor on the constitutively activated signalling pathway, and provides a framework to understand and evaluate the effect of anticancer drugs on tumour cells. Then, we asked whether a similar decrease in sensitivity to an inhibitor could occur under such conditions. We found that Z peak was similarly less sensitive to the inhibitor than Y peak under physiologically relevant conditions ( Supplementary Fig. S8 ). This finding raises the possibility that the downstream molecule may be less sensitive to an inhibitor than the target molecule in vivo . We examined the conditions for the attenuation of signal transfer efficiency in the activator model ( Fig. 7a ) and found that the signal transfer efficiency is attenuated when the duration of upstream signal, t 1/2 , is shorter than the time constant of negative regulation, τ . Thus, the attenuation of signal transfer efficiency can be controlled by negative regulation ( Fig. 7b ). We found experimentally that the attenuation of signal transfer efficiency is a conserved property of linear signalling pathways, regardless of the specific pathways, growth factors and cell lines. 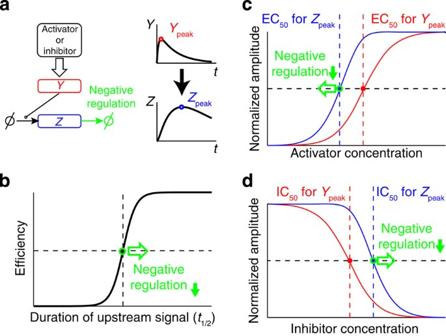Figure 7: Negative regulation controls the signal transfer efficiency and sensitivity to an activator or an inhibitor. (a) Conceptual description of the activator and inhibitor model. The negative regulation ofZmay correspond to the degradation or dephosphorylation of a signalling pathway. (b) Attenuation of the signal transfer efficiency by negative regulation. The weaker the negative regulation becomes, the stronger the attenuation of efficiency becomes. (c) Control of sensitivity to an activator by negative regulation. The weaker the negative regulation becomes, the more sensitive the downstream molecule becomes. (d) Control of sensitivity to an inhibitor by negative regulation. The weaker the negative regulation becomes, the less sensitive the downstream molecule becomes. Figure 7: Negative regulation controls the signal transfer efficiency and sensitivity to an activator or an inhibitor. ( a ) Conceptual description of the activator and inhibitor model. The negative regulation of Z may correspond to the degradation or dephosphorylation of a signalling pathway. ( b ) Attenuation of the signal transfer efficiency by negative regulation. The weaker the negative regulation becomes, the stronger the attenuation of efficiency becomes. ( c ) Control of sensitivity to an activator by negative regulation. The weaker the negative regulation becomes, the more sensitive the downstream molecule becomes. ( d ) Control of sensitivity to an inhibitor by negative regulation. The weaker the negative regulation becomes, the less sensitive the downstream molecule becomes. Full size image We also found that the downstream molecule was more sensitive to activators than the upstream molecule. This increase in the downstream sensitivity to the activator can be controlled by negative regulation by the attenuation of signal transfer efficiency ( Fig. 7c ). Similarly, the downstream molecule was less sensitive to inhibitors than the upstream molecule, and this can also be controlled by negative regulation by the attenuation of signal transfer efficiency ( Fig. 7d ). The decrease in the sensitivity of the downstream molecule to an inhibitor was verified experimentally. We also found that the downstream molecule was less sensitive to the inhibitor than the upstream molecule under physiologically relevant conditions, where upstream molecules are constitutively active. The sensitivities of the molecules to an activator or an inhibitor depended on the rate constant of negative regulation. The attenuation of signal transfer efficiency by negative regulation is one of the core mechanisms to control sensitivity to activators and inhibitors. Negative regulation, conditions about the analysis of sensitivity control, comparing with previous studies about sensitivity and extent of the attenuation of signal transfer efficiency are discussed in Supplementary Note 2 . Cell culture and growth factor treatments Cell culture and growth factor stimulation were performed as previously described [23] . Briefly, PC12 cells were provided by M. Nakafuku (Cincinnati Children's Hospital Medical Center, Cincinnati, OH) and cultured in Dulbecco's modified Eagle's medium (low-glucose, Sigma, #D6046) supplemented with 10% fetal bovine serum (FBS) and 5% horse serum. The PC12 cells (8×10 5 cells) were seeded onto 60-mm poly- D -lysine-coated dishes. One day later, the PC12 cells were serum starved for 16 h and then stimulated with EGF or NGF, as previously described [23] . In the inhibitor experiment, lapatinib (Toronto Research Chemicals, #L175800) was added from serum starvation, and the cells were stimulated with EGF (30 ng ml −1 ; Fig. 6 ). The HeLa cells were kindly provided by S. Sigismund (Fondazione Istituto FIRC di Oncologia Molecolare, Milan, Italy) [24] and cultured in minimum essential medium (Sigma, #M4655) supplemented with 10% FBS, 1 mM sodium pyruvate and 0.1 mM MEM non-essential amino acids (Invitrogen, #11140-050). The HeLa cells (2×10 5 cells) were seeded onto 60-mm poly- D -lysine-coated dishes. One day later, the medium in which the HeLa cells were grown was renewed, and after 16 h the HeLa cells were stimulated with EGF (0, 1 or 100 ng ml −1 ). Swiss-3T3 cells were obtained from the Health Science Research Resources Bank (Osaka, Japan, #JCRB9019) and cultured in Dulbecco's modified Eagle's medium (low-glucose, Sigma #D6046) supplemented with 10% FBS. The Swiss-3T3 cells (1.5×10 5 cells) were seeded onto 35-mm non-treated dishes. Two days later, the Swiss-3T3 cells were serum starved for 16 h and then stimulated with EGF (0.1, 1, 10 and 100 ng ml −1 ) [25] . The HUVECs and culture media (HuMedia-EG2) were purchased from a commercial source (Kurabo) [26] . The HUVECs (3×10 5 cells) at the sixth passage were seeded onto 35-mm collagen-coated dishes. One day later, the HUVECs were serum starved for 16 h and then stimulated with EGF (0.1, 0.3, 1, 3, 10, 30 and 100 ng ml −1 ) [27] . Immunoblotting Immunoblotting and the processing of the signal intensities of the immunoblots were performed as previously described [23] . All antibodies were purchased from Cell Signaling Technology, as follows: PathScan Multiplex Western Cocktail I (antibodies against phosphorylated p90RSK (Ser380), phosphorylated Akt (Ser473), phosphorylated ERK1/2 (Thr202/Tyr204), phosphorylated S6 (Ser235/236) and total eIF4E, #5301), phosphorylated EGFR (Tyr1068) (#2234), phosphorylated TrkA (Tyr490) (#9141), phosphorylated TSC2 (Thr1462) (#3617), phosphorylated S6 kinase (Thr389) (#9205 or #9206), phosphorylated eIF4B (Ser422) (#3591), phosphorylated GSK3β (Ser9) (#9336), phosphorylated CREB (Ser133) (#9191), c-Fos (#2250), c-Jun (#9165), EGR1 (#4154) and p21Cip1 (#2947). The immunoblotting was performed using Immobilon Western Chemiluminescent HRP Substrate (Millipore), and the immunoblot signals were detected using a luminoimage analyser (LAS-4000; Fujifilm). A portion of the experimental data shown in Figs 3 and 6 represent previously reported data [23] . Simulation and parameter estimation We performed the simulation and analysis using MATLAB (version R2010a, MathWorks) and SBTOOLBOX2 [28] , a third-party toolbox for MATLAB. We estimated the parameters based on a previously reported protocol [23] . Details of the parameter estimation method are described in Supplementary Note 1 . Experimental validation of the attenuation property We obtained 568 sets of time courses of 110 pathways from the experiments in four cell lines stimulated by two ligands ( Supplementary Data 2 ). Each pathway consists of an upstream and a downstream molecule. When the cell lines, ligand or stimulation pattern (step, pulse or ramp stimulation) is different, the same set of upstream and downstream molecules is regarded as a different pathway. For each pathway, time courses were obtained using multiple doses. We estimated the parameters of the activator model for each set of experimental time courses (see Supplementary Note 1 and Supplementary Data 2 ). The values of c and d were estimated for each pathway because c and d were constant for a given pathway and should be conserved, regardless of the dose of a stimulating ligand applied, whereas a and b were estimated for each dose of stimulation because a and b were parameters for stimulation, and could vary depending on the dose applied. We selected pathways that satisfied conditions (a) and (b) (see Supplementary Note 2 ) as follows. The squared sum of the residuals (RSS) between experiment and simulation were calculated for each time course or for all time courses in each pathway, and then normalized by the squared sum of the experimental value. We excluded the pathways for which the normalized RSS was >0.1 and the set of time courses for which the normalized RSS was >0.3. We also excluded the time courses of the inhibitor experiments and the set of time courses for which the duration of upstream signal ( t 1/2 ) or the peak amplitudes could not be obtained experimentally because of the sustained response or nonresponse to the stimuli. We selected the rest of the time courses as satisfying conditions (a) and (b), and analysed the corresponding experimental data to produce Fig. 3 . The duration of upstream signal ( t 1/2 ) was obtained by linear interpolation of the experimental time course of the upstream molecule. The signal transfer efficiency ( E ) was obtained from the ratio of the peak amplitudes of the experimental time courses and then normalized by the gain of the fitted activator model. How to cite this article: Toyoshima, Y. et al . Sensitivity control through attenuation of signal transfer efficiency by negative regulation of cellular signalling. Nat. Commun. 3:743 doi: 10.1038/ncomms1745 (2012).